Structural basis for catalysis in a CDP-alcohol phosphotransferase The CDP-alcohol phosphotransferase (CDP-AP) family of integral membrane enzymes catalyses the transfer of a substituted phosphate group from a CDP-linked donor to an alcohol acceptor. This is an essential reaction for phospholipid biosynthesis across all kingdoms of life, and it is catalysed solely by CDP-APs. Here we report the 2.0 Å resolution crystal structure of a representative CDP-AP from Archaeoglobus fulgidus. The enzyme (AF2299) is a homodimer, with each protomer consisting of six transmembrane helices and an N-terminal cytosolic domain. A polar cavity within the membrane accommodates the active site, lined with the residues from an absolutely conserved CDP-AP signature motif (D 1 xxD 2 G 1 xxAR…G 2 xxxD 3 xxxD 4 ). Structures in the apo, CMP-bound, CDP-bound and CDP-glycerol-bound states define functional roles for each of these eight conserved residues and allow us to propose a sequential, base-catalysed mechanism universal for CDP-APs, in which the fourth aspartate (D 4 ) acts as the catalytic base. A key step in the synthesis of most phospholipids in both eukaryotes [1] and prokaryotes [2] , [3] involves the transfer of a substituted phosphate group from a CDP-linked donor to an acceptor alcohol to generate a phosphodiester-linked product. This essential reaction for the formation of phospholipid bilayers is catalysed exclusively by a family of membrane-embedded enzymes known as CDP-alcohol phosphotransferases (CDP-APs). CDP-APs facilitate the conjugation of a polar headgroup, such as choline, inositol or ethanolamine, to a diacylglycerol lipid tail, resulting in the formation of polar phospholipids such as phosphatidylcholine (PC), phosphatidylinositol (PI) and phosphatidylethanolamine (PE). 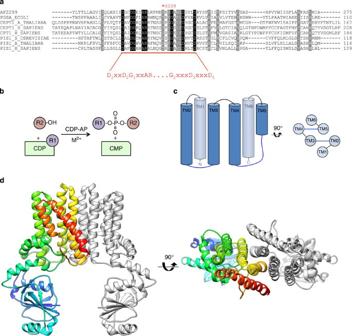Figure 1: The structure of AF2299 reveals the architecture of a CDP-alcohol phosphotransferase. (a) The CDP-AP signature motif is absolutely conserved across all kingdoms of life. Alignment of eight CDP-APs of divergent sequence shows that the CDP-AP signature motif (D1xxD2G1xxAR…G2xxxD3xxxD4) is absolutely conserved, and is present in AF2299. Alignment performed using PROMALS3D48. Sequences, from top, (as species—protein; Uniprot ID) are:A. fulgidus—AF2299; O27985,E. coli—PGP synthase PgsA; P0ABF8,A. thaliana—choline/ethanolamine phosphotransferase; O82567,H. sapiens—choline/ethanolamine phosphotransferase; Q9Y6K0,H. sapiens—choline phosphotransferase; Q8WUD6,S. cerivisiae—phosphatidylinositol synthase; P06197,A. thaliana—phosphatidylinositol synthase; Q8LBA6,H. sapiens—phosphatidylinositol synthase; O14735. (b) CDP-alcohol phosphotransferases catalyse the transfer of a phosphate group, with donor substituent R1 (where R1 may represent choline, ethanolamine, or diacylglycerol, amongst others) to an alcohol, with substituent R2 (where R2 may represent inositol, inositol-1-phosphate, glycerol-3-phosphate choline or diacylglycerol, for example). (c) Each subunit of AF2299 possesses six TM helices arranged in two repeats of three. TM5 is noticeably shorter than the rest. Intracellular loops are represented by blue lines and extracellular loops by black lines. The juxtamembrane helix and N-terminal domain are not shown. The left half of this panel is represented in an open form such that the two repeats are side by side. (d) AF2299 is a dimer of two subunits each with six TM helices and an N-terminal domain of the cytidyltransferase fold. The protein is depicted with one subunit in grey and the other in rainbow coloured ribbon representation, from blue (N terminus) to red (C terminus), viewed (on the left) in the plane of the membrane, and (on the right) from the extracellular side of the membrane down the dimer interface. Depending on the enzyme and on organism, the diacylglycerol tail or the polar headgroup may participate as either the CDP-linked donor substrate, or the acceptor alcohol ( Supplementary Table 1 ). Furthermore, both substrates may be lipids, as in cardiolipin synthase [4] , or polar small molecules [5] , further exemplifying the broad substrate specificity of this diverse class of enzymes for which the only two required elements are a terminal hydroxyl on the acceptor and a CDP-linkage on the donor. CDP-APs exhibit broad variety in the identity and lipophilic versus hydrophilic nature of the acceptor and donor substrates they process. Irrespective of the identity of the substrates, they are all predicted to be integral membrane proteins and possess a universally conserved signature motif of eight amino acids spaced over a small stretch of sequence (D 1 xxD 2 G 1 xxAR…G 2 xxxD 3 xxxD 4 ; Fig. 1a,b ). The absolute conservation of the signature motif in enzymes with such diverse substrate specificities suggests that it plays a fundamental role in catalysing phosphotransfer, but the absence of any structural information has hampered progress in understanding the mechanism of this essential class of integral membrane enzymes. Here we report the structure of AF2299, a representative CDP-AP from Archaeoglobus fulgidus , revealing the transmembrane (TM) architecture of an integral membrane phosphotransferase, unveiling the role of each conserved residue in the signature motif in the reaction, and allowing us to postulate a universal mechanism of catalysis for this reaction. Figure 1: The structure of AF2299 reveals the architecture of a CDP-alcohol phosphotransferase. ( a ) The CDP-AP signature motif is absolutely conserved across all kingdoms of life. Alignment of eight CDP-APs of divergent sequence shows that the CDP-AP signature motif (D 1 xxD 2 G 1 xxAR…G 2 xxxD 3 xxxD 4 ) is absolutely conserved, and is present in AF2299. Alignment performed using PROMALS3D [48] . Sequences, from top, (as species—protein; Uniprot ID) are: A. fulgidus— AF2299; O27985, E. coli —PGP synthase PgsA; P0ABF8, A. thaliana— choline/ethanolamine phosphotransferase; O82567, H. sapiens— choline/ethanolamine phosphotransferase; Q9Y6K0, H. sapiens— choline phosphotransferase; Q8WUD6, S. cerivisiae— phosphatidylinositol synthase; P06197, A. thaliana— phosphatidylinositol synthase; Q8LBA6, H. sapiens— phosphatidylinositol synthase; O14735. ( b ) CDP-alcohol phosphotransferases catalyse the transfer of a phosphate group, with donor substituent R1 (where R1 may represent choline, ethanolamine, or diacylglycerol, amongst others) to an alcohol, with substituent R2 (where R2 may represent inositol, inositol-1-phosphate, glycerol-3-phosphate choline or diacylglycerol, for example). ( c ) Each subunit of AF2299 possesses six TM helices arranged in two repeats of three. TM5 is noticeably shorter than the rest. Intracellular loops are represented by blue lines and extracellular loops by black lines. The juxtamembrane helix and N-terminal domain are not shown. The left half of this panel is represented in an open form such that the two repeats are side by side. ( d ) AF2299 is a dimer of two subunits each with six TM helices and an N-terminal domain of the cytidyltransferase fold. The protein is depicted with one subunit in grey and the other in rainbow coloured ribbon representation, from blue (N terminus) to red (C terminus), viewed (on the left) in the plane of the membrane, and (on the right) from the extracellular side of the membrane down the dimer interface. Full size image Structure determination To understand the structural basis for catalysis in CDP-APs we determined crystal structures of AF2299, a representative member of this family from Archaeoglobus fulgidus , in the apo form, with bound CDP, and with bound CMP. The crystals, grown from lipidic cubic phase, belong to space group P 2 1 with one homodimer per asymmetric unit, and they diffract X-rays to 1.9 Å (CMP/apo) and 2.1 Å (CDP) respectively. We report two structures, one with both active sites occupied by CDP (PDB accession number 4O6N ), and the other with one active site bound by CMP and the other one in the apo state (PDB accession number 4O6M ). Both structures were obtained with co-purified ligands. To shed light on the key elements for substrate specificity, we also determined the structure to 3.1 Å resolution of AF2299 co-crystallized with CDP-glycerol, the likely donor substrate for this enzyme. Architecture of a CDP-alcohol phosphotransferase AF2299 is a homodimer, with each protomer consisting of two distinct domains. An N-terminal cytoplasmic domain of unknown function has clear structural similarity to the cytidyltransferases [6] , but the active site residues are not conserved, suggesting that it may lack catalytic activity. The cytidyltransferase domain perhaps represents an evolutionary vestige of a bifunctional enzyme that performed the function of generating the CDP-donor substrate in addition to the phosphotransferase activity retained in AF2299. Such dual-function enzymes have been characterized in archaea [7] . The N-terminal cytidyltransferase domain is followed by a C-terminal TM domain consisting of six TM helices arranged as two inverted repeats of three helices ( Figs 1c,d and 2a ). The dimer interface is symmetric, and involves TM 3 and TM 4 ( Fig. 2a ). All TM helices except TM5 extend beyond the predicted intracellular surface of the membrane by three to four turns ( Fig. 2b ). A curved juxtamembrane helix wraps around the outer surface of TM2 and TM5. A mobile loop (ordered in only one of the two subunits) provides a connection between the last helix of the cytidyltransferase domain and the juxtamembrane helix ( Fig. 1d ). 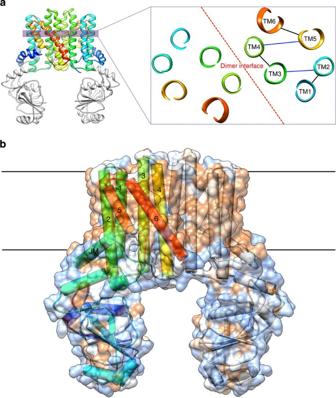Figure 2: Architecture of the AF2299 dimer. (a) Two inverted repeats of three helices (TM1-3 and TM4-6) surround a central cavity in each monomer. The dimer interface is formed by TM 3 and 4, and buries an area of 1,963 Å2. Here, on the left, a dimer is represented with the N-terminal domains in grey and the TM subunits in rainbow ribbon representation, from blue (N-terminal) to red (C-terminal). A 4 Å thick slab (purple shading) is withdrawn from the protein, and on the right, viewed from the extracellular side of the membrane down the dimer interface (red dashed line). The helices are labelled TM1–TM6, and connections between them are represented either in black (for extracellular loops) or blue (for intracellular loops). (b) All TM helices except TM5 extend beyond the intracellular border of the membrane. Here, the TM helices of AF2299 are represented as cylinders, and the secondary structure elements of the protomer on the left are coloured in rainbow representation, from blue (N terminus) to red (C terminus). The TM helices are labelled from 1 to 6. The dimer is represented inside a translucent molecular surface coloured by the Kyte–Doolitle hydrophobicity scale from −4.5 (most polar, light blue) to 4.5 (most hydrophobic, orange). The approximate boundaries of the membrane are represented by black lines. Figure 2: Architecture of the AF2299 dimer. ( a ) Two inverted repeats of three helices (TM1-3 and TM4-6) surround a central cavity in each monomer. The dimer interface is formed by TM 3 and 4, and buries an area of 1,963 Å 2 . Here, on the left, a dimer is represented with the N-terminal domains in grey and the TM subunits in rainbow ribbon representation, from blue (N-terminal) to red (C-terminal). A 4 Å thick slab (purple shading) is withdrawn from the protein, and on the right, viewed from the extracellular side of the membrane down the dimer interface (red dashed line). The helices are labelled TM1–TM6, and connections between them are represented either in black (for extracellular loops) or blue (for intracellular loops). ( b ) All TM helices except TM5 extend beyond the intracellular border of the membrane. Here, the TM helices of AF2299 are represented as cylinders, and the secondary structure elements of the protomer on the left are coloured in rainbow representation, from blue (N terminus) to red (C terminus). The TM helices are labelled from 1 to 6. The dimer is represented inside a translucent molecular surface coloured by the Kyte–Doolitle hydrophobicity scale from −4.5 (most polar, light blue) to 4.5 (most hydrophobic, orange). The approximate boundaries of the membrane are represented by black lines. Full size image CDP binds within a cavity lined by the signature motif The six TM helices of AF2299 surround a polar, positively charged cavity extending from the cytosol to a depth of 8 Å into the membrane ( Fig. 3a and Supplementary Fig. 1 ). The CDP-AP signature motif lines one side of this polar cavity formed by the cytosolic ends of TM2 and TM3, and defines the active site ( Fig. 3b,c ). The two conserved segments of the motif reside on TM2 and TM3 respectively, and the residues that separate them constitute the loop joining the two TM helices ( Fig. 3c ). Of the four conserved aspartic acid residues in the signature motif, the first (D 1 , Asp214) and the second (D 2 , Asp217) on TM2 directly face the fourth (D 4 , Asp239) and the third (D 3 , Asp235) respectively on TM3 ( Fig. 3b ). The first conserved glycine (G 1 , Gly218) provides the necessary flexibility to TM2 to allow the carbonyl of D 1 to reorient away from the helix axis towards the active site. In the structures with bound CDP or CMP, the ligand is wedged in a cleft between TM2 and TM3, and backed by TM1 ( Fig. 3c and Supplementary Fig. 2 ). The conserved alanine (Ala221) and G 1 interact with one face of the planar cytosine ring while the second conserved glycine (G 2 , Gly231) interacts with the opposite face. The N-terminal end of TM1 also contributes to nucleotide binding, primarily through interactions of a small segment that includes a conserved threonine (Thr178) that forms part of a hydrogen bonding network stabilizing the polar edge of the cytosine ring ( Supplementary Fig. 3a,b ). The invariant arginine (Arg222) interacts with the α-phosphate of CDP, and this interaction is retained in the CMP-bound state ( Supplementary Fig. 3a,b ). Finally, it may be worth mentioning that Ser228, another residue in this network, forms a water-mediated hydrogen bond to N3 in the pyrimidine ring. This residue is typically either a serine or threonine in CDP-APs ( Fig. 1a ), and a well-characterized mutation (T60P) of the equivalent residue in the E. coli gene PgsA, which encodes a phosphatidylglycerophosphate (PGP) synthase, results in a defect in phosphatidylglycerol synthesis [8] , [9] . 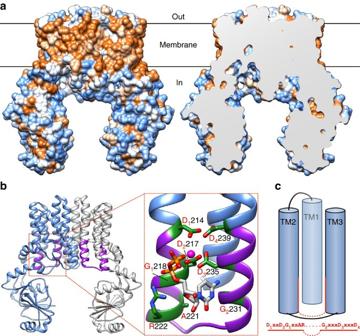Figure 3: The signature motif of the CDP-alcohol phosphotransferase family is located around a cleft between TM helices 2 and 3. (a) Each subunit possesses a polar cavity near the surface of the membrane. Here, the molecular surface of AF2299 is coloured by Kyte–Doolitle hydrophobicity49from −4.5 (most polar, light blue) to 4.5 (most hydrophobic, orange). On the right, the front half of the dimer has been removed to expose the polar cavities in each subunit that penetrate 8 Å beyond the intracellular border of the membrane. The approximate borders of the membrane, as calculated by the PPM server50, are indicated by black lines. (b) The CDP-alcohol phosphotransferase signature motif spans the cytosolic ends of TM2 and TM3 (highlighted here in purple; the conserved residues of the signature motif are shown in green stick representation in a zoom-in panel on the right, as is the CDP (in grey stick) and the primary divalent cation (as a pink sphere). (c) TM 2 and 3 (blue cylinders) form a groove, backed by TM1, lined by the residues of the signature motif (solid red line; the non-conserved segment between the two helices is indicated by a dashed red line). Figure 3: The signature motif of the CDP-alcohol phosphotransferase family is located around a cleft between TM helices 2 and 3. ( a ) Each subunit possesses a polar cavity near the surface of the membrane. Here, the molecular surface of AF2299 is coloured by Kyte–Doolitle hydrophobicity [49] from −4.5 (most polar, light blue) to 4.5 (most hydrophobic, orange). On the right, the front half of the dimer has been removed to expose the polar cavities in each subunit that penetrate 8 Å beyond the intracellular border of the membrane. The approximate borders of the membrane, as calculated by the PPM server [50] , are indicated by black lines. ( b ) The CDP-alcohol phosphotransferase signature motif spans the cytosolic ends of TM2 and TM3 (highlighted here in purple; the conserved residues of the signature motif are shown in green stick representation in a zoom-in panel on the right, as is the CDP (in grey stick) and the primary divalent cation (as a pink sphere). ( c ) TM 2 and 3 (blue cylinders) form a groove, backed by TM1, lined by the residues of the signature motif (solid red line; the non-conserved segment between the two helices is indicated by a dashed red line). Full size image Divalent cation-binding sites All CDP-APs require a divalent cation for activity, most often Mg 2+ (ref. 10 ), Mn 2+ (ref. 11 ), or Co 2+ (ref. 12 ). In the structure of AF2299, a bound metal ion mediates the interaction of the pyrophosphate moiety of CDP with the sidechains of D 2 and D 3 , and with the backbone carbonyl of D 1 ( Fig. 3b ). In the CDP-bound and apo structures only, a secondary metal binding site is located 4 Å away from the first, coordinated by the side chains of D 1 , D 3 and D 4 ( Supplementary Fig. 3c ). We could not observe any anomalous signal derived from these ions, a strong indication that points to the exclusion of transition metals, leaving Ca 2+ or Mg 2+ as possibilities. Details of their coordination are most consistent with Ca 2+ , due to both the pentagonal–bipyramid coordination geometry and bond distances in the range of 2.3–2.7 Å, which are considerably longer than would be expected for Mg 2+ ions [13] . We confirmed the identity of the divalent cations as Ca 2+ by flame atomic absorption spectrophotometry on purified protein. Indeed, by this method we could measure a signal from Ca above background and equimolar to the concentration of AF2299 (Methods and Supplementary Table 2 ), while we could not detect the presence of any protein-associated Mg. Two substrate-binding pockets are located within the polar cavity Deeper in the active site of the CMP and apo structures, a tetrahedral oxyanion, probably sulphate given its presence in the crystallization solution, is bound by Arg240 and Arg304 ( Fig. 4a and Supplementary Fig. 3d ). The sulphate also forms a hydrogen bond with the amide nitrogen of Arg301, which lies at the N-terminal end of the short TM5, consistent with a role for the helix dipole in stabilization of anion binding [14] . The oxyanion-binding site is formed by residues that are conserved in a manner that appears to correlate with the identity of the acceptor. In the CDP structure, for which tartrate rather than sulphate was present in the crystallization solution, a tartrate ion is found in the same position occupied by the sulphate in the CMP and apo structures ( Supplementary Fig. 4 ). Sequence analysis reveals that Arg240 is conserved in all enzymes that take either inositol or inositol phosphate as the acceptor and that a short motif (R 301 xxR 304 , in AF2299 numbering) is specifically conserved in the subset of these enzymes that utilize inositol-1-phosphate ( Fig. 4b,c ). We hypothesize that Arg240 forms hydrogen bonds with hydroxyls 2/3 or 5/6 of the inositol, fixing the orientation of the ring in a catalytically competent orientation, with the 4-OH positioned in-line with the pyrophosphate moiety of the CDP-donor. The data that we present here are insufficient to assign the identity of the acceptor alcohol for AF2299; however, they do allow us to identify with reasonable certainty the location of the acceptor binding-site, which we would expect to be conserved throughout the family of CDP-APs. 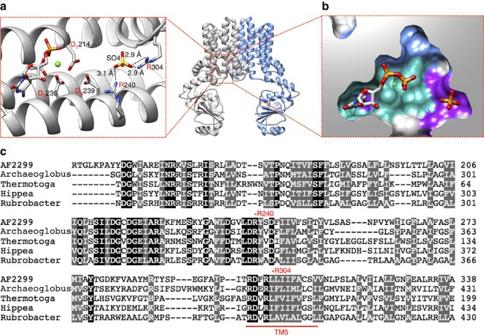Figure 4: Two binding pockets within the cavity form putative binding sites for the donor subtituent and the acceptor alcohol. (a) The putative catalytic aspartate, D239, lies approximately equidistant between the bound CMP and a bound sulphate ion, located between two arginine residues, R240 and R304. (b) Family-specific conservation patterns delineate three regions within the cavity. Residues conserved in all members of the CDP-alcohol phosphotransferase family are coloured in cyan, those conserved only in enzymes that utilize inositol-1-phosphate as an acceptor are coloured in purple, and those that are conserved in all enzymes known to bind CDP-inositol or CDP-glycerol in light blue. The bound sulphate and CDP are shown in stick representation. (c) An alignment of AF2299 with DIPP synthases shows several highly conserved regions outside the signature motif; notably, the two arginines that coordinate the bound sulfate, R240 and R304 (indicated in red), are absolutely conserved. Figure 4: Two binding pockets within the cavity form putative binding sites for the donor subtituent and the acceptor alcohol. ( a ) The putative catalytic aspartate, D239, lies approximately equidistant between the bound CMP and a bound sulphate ion, located between two arginine residues, R240 and R304. ( b ) Family-specific conservation patterns delineate three regions within the cavity. Residues conserved in all members of the CDP-alcohol phosphotransferase family are coloured in cyan, those conserved only in enzymes that utilize inositol-1-phosphate as an acceptor are coloured in purple, and those that are conserved in all enzymes known to bind CDP-inositol or CDP-glycerol in light blue. The bound sulphate and CDP are shown in stick representation. ( c ) An alignment of AF2299 with DIPP synthases shows several highly conserved regions outside the signature motif; notably, the two arginines that coordinate the bound sulfate, R240 and R304 (indicated in red), are absolutely conserved. Full size image Another apparent binding pocket extends into the wall of the polar cavity, perpendicular to the CDP pyrophosphate ( Fig. 4b ). This site is lined by residues specifically conserved in the archaeal family of CDP-APs that utilize donors with small, polar substituents, such as CDP-inositol and CDP-glycerol, to generate soluble phosphodiester-linked osmolytes that apparently help their host organisms endure thermal and osmotic stress [15] . This family includes the di-myo-inositol-1,3′-phosphate-1′- phosphate synthase (DIPPS) subfamily of CDP-APs, which are the best-characterized enzymes of this class [16] . Based on this observation, we suggest that this pocket may accommodate the donor substituent, and that AF2299 may catalyse the reaction of inositol-1-phosphate with a small molecule, possibly CDP-glycerol or CDP-inositol [5] . Indeed, co-crystallization with CDP-glycerol reveals additional density in this pocket consistent with binding of the glycerol moiety ( Fig. 5 ). This is in agreement with the observation that the AF2299 sequence is most closely related to those of the DIPPS family ( Figs 4c and 6 ). Given our structure with bound CDP-glycerol and the fact that an A. fulgidus DIPPS enzyme (AF0263) has already been identified [7] , the most plausible hypothesis is that AF2299 catalyses the condensation of CDP-glycerol with L- myo -inositol-1-phosphate, to yield the glyceryl phosphodiester of inositol-1-phosphate, although experimental confirmation of this conjecture awaits further studies. 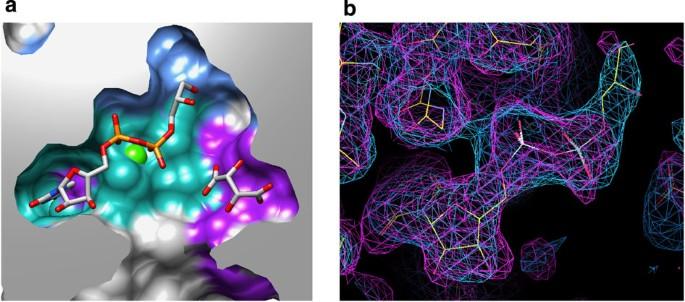Figure 5: Binding of CDP-glycerol in the active site. (a) A co-crystal structure with CDP-glycerol reveals that the glycerol moiety binds in the putative donor-substituent binding pocket (Colors as forFig. 4). (b) 2Fo−Fcomit maps (calculated prior to ligand placement) contoured at 1σfor the CDP and CDP-glycerol structures are represented as purple and blue mesh, respectively. The CDP-glycerol ligand from the final refined structure is depicted in stick representation. Figure 5: Binding of CDP-glycerol in the active site. ( a ) A co-crystal structure with CDP-glycerol reveals that the glycerol moiety binds in the putative donor-substituent binding pocket (Colors as for Fig. 4 ). ( b ) 2F o −F c omit maps (calculated prior to ligand placement) contoured at 1 σ for the CDP and CDP-glycerol structures are represented as purple and blue mesh, respectively. The CDP-glycerol ligand from the final refined structure is depicted in stick representation. 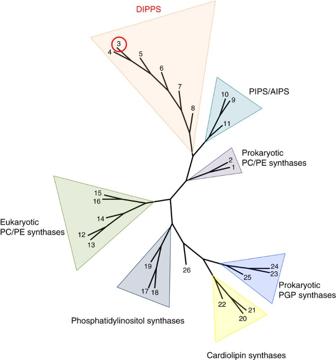Figure 6: AF2299 is most closely related in sequence to the di-inositol-phosphate synthases. AF2299 (3, highlighted by a red circle), is most similar in sequence to the previously characterized DIPP synthases (4–8). Here, an unrooted phylogenetic tree, generated using CLUSTALW-PHYLOGENY51from a multiple-alignment of 26 sequences (performed using CLUSTAL-OMEGA52), was visualized in radial representation using T-REX53, and manually edited for clarity. The sequences cluster into distinct families of related function (shaded triangles), and AF2299 is most closely related to those that have been functionally characterized as DIPP synthases (orange shaded triangle). The species and Uniprot IDs of the sequences used to generate the tree are as follows: (1) Q9KJY8;Rhizobium meliloti.(2): Q98MN3;Rhizobium loti.(3) O27985;Archeoglobus fulgidus(AF2299). (4) O29976;Archaeoglobus fulgidus.(5) Q5JDA9;Thermococcus kodakaraensis.(6) Q8U1Z6;Pyrococcus furiosus. (7) O67379;Aquafex aeolicus.(8) Q1AWQ0;Rubrobacter xylanophilus.(9) O27726;Methanothermobacter thermautotrophicus. (10) Q9F7Y9;Mycobacterium smegmatis.(11) Q7D6W6;Mycobacterium tuberculosis. (12) Q8WUD6;Homo sapiens.(13) Q5ZKD1;Gallus gallus.(14) Q9Y6K0;Homo sapiens. (15) P17898;Saccharomyces cerevisiae.(16) O82567;Arabidopsis thaliana.(17) Q8LBA6;Arabidopsis thaliana.(18) P06197;Saccharomyces cerevisiae.(19) O14735;Homo sapiens.(20) Q8MZC4;Drosophila melanogaster.(21) Q9UJA2;Homo sapiens.(22) O01916;Caenorhabditis elegans. (23) Q68XS5;Ricksettia typhi.(24) P0ABF8;Escherichia coli. (25) P44528;Haemophilus influenza.(26) P63753;Mycobacterium tuberculosis. Full size image Figure 6: AF2299 is most closely related in sequence to the di-inositol-phosphate synthases. AF2299 (3, highlighted by a red circle), is most similar in sequence to the previously characterized DIPP synthases (4–8). Here, an unrooted phylogenetic tree, generated using CLUSTALW-PHYLOGENY [51] from a multiple-alignment of 26 sequences (performed using CLUSTAL-OMEGA [52] ), was visualized in radial representation using T-REX [53] , and manually edited for clarity. The sequences cluster into distinct families of related function (shaded triangles), and AF2299 is most closely related to those that have been functionally characterized as DIPP synthases (orange shaded triangle). The species and Uniprot IDs of the sequences used to generate the tree are as follows: (1) Q9KJY8; Rhizobium meliloti. (2): Q98MN3; Rhizobium loti. (3) O27985; Archeoglobus fulgidus (AF2299). (4) O29976; Archaeoglobus fulgidus. (5) Q5JDA9; Thermococcus kodakaraensis. (6) Q8U1Z6; Pyrococcus furiosus . (7) O67379; Aquafex aeolicus. (8) Q1AWQ0; Rubrobacter xylanophilus. (9) O27726; Methanothermobacter thermautotrophicus . (10) Q9F7Y9; Mycobacterium smegmatis. (11) Q7D6W6; Mycobacterium tuberculosis . (12) Q8WUD6; Homo sapiens. (13) Q5ZKD1; Gallus gallus. (14) Q9Y6K0; Homo sapiens . (15) P17898; Saccharomyces cerevisiae. (16) O82567; Arabidopsis thaliana. (17) Q8LBA6; Arabidopsis thaliana. (18) P06197; Saccharomyces cerevisiae. (19) O14735; Homo sapiens. (20) Q8MZC4; Drosophila melanogaster. (21) Q9UJA2; Homo sapiens. (22) O01916; Caenorhabditis elegans . (23) Q68XS5; Ricksettia typhi. (24) P0ABF8; Escherichia coli . (25) P44528; Haemophilus influenza. (26) P63753; Mycobacterium tuberculosis. Full size image The structure of AF2299 reveals that CDP-APs adopt what is, to the best of our knowledge, a novel fold, with six TM helices surrounding a polar cavity. The active site of AF2299 is located near the surface of the membrane with direct access to the cytosol, consistent with the function of many CDP-APs in binding one soluble and one membrane-embedded substrate. It is tempting to speculate that the gap in the wall of the polar cavity created by the shorter TM5 helix may facilitate access of CDP-linked lipids to the active site, in those enzymes that utilize CDP-archaeol or CDP-diacylglycerol as donor substrates. Access of CDP-linked lipids by such a route would not be possible in AF2299 from our current structures, as the N-terminal end of the juxtamembrane helix occludes this hypothetical pathway, but only a slight alteration in the length or conformation of this helix would be necessary to facilitate lipid binding. Sequence alignment and secondary structure prediction for other CDP-alcohol phosphotransferases suggests that at least the PI-synthases share the same fold as the TM domain of AF2299, with an amphipathic juxtamembrane helix followed by six TM helices, of which the fifth is considerably shorter than the other five ( Supplementary Fig. 5 ). Interestingly, enzymes that utilize a lipid acceptor, such as the eukaryotic phosphatidylcholine synthases, which take CDP-choline as a donor and diacylglycerol as an acceptor, have a somewhat different architecture, characterized by the presence of an additional 3–4 TM helices at the C terminus, perhaps in order to accommodate the bulkier lipid acceptor. The membrane localization of CDP-APs such as AF2299 and the DIPP synthases, which condense two soluble substrates, is intriguing and we suggest that it may have an evolutionary explanation. If the ancestral proto-CDP-AP from which all current CDP-APs are derived was an integral membrane protein with hydrophobic substrates, it is difficult to envision how the enzyme architecture could be modified during evolution to become a soluble protein, but it is not unlikely that slight modifications around the active site could result in entry of and affinity for a pair of soluble substrates. The structures of AF2299 in the apo, CMP-bound and CDP-bound forms presented here provide us with the opportunity to dissect the structural basis for catalysis in a CDP-AP. It has been suggested that reactions catalysed by CDP-APs proceed by a sequential mechanism involving a nucleophilic attack of the acceptor on the β-phosphorous of the CDP-donor [17] , [18] , but the roles of residues in the signature motif have remained unclear, although it has been previously suggested that either D 3 or D 4 may act as a catalytic base [19] . The AF2299 structures reveal that D 1 , D 2 and D 3 coordinate the pyro-phosphate of CDP via the primary divalent cation. D 4 , in contrast, based on its position approximately equidistant between the acceptor and donor binding sites ( Supplementary Fig. 4 ), is likely to play a key role in catalysis. In S. cerevisiae choline phosphotransferase, mutation of the equivalent residue results in complete abolition of enzymatic activity [19] . Likewise, mutation of D 4 in an aminoalcoholphosphotransferase from Brassica napus (rapeseed) results in the loss of detectable phosphotransferase activity [20] . A more extensive alanine mutagenesis scan in Rhizobium meliloti phosphatidylcholine synthase yielded the same conclusions [21] . Furthermore, D 4 does not interact with the CDP either directly or via the bridging divalent cation. In summary, D 4 is absolutely conserved, essential for activity in enzymes from two different kingdoms ( Plantae and Fungi ), but does not appear to participate in substrate binding, and is located between the binding sites of the acceptor and donor substrates. These observations support a direct role for D 4 in the mechanism of phosphotransfer in CDP-APs. We propose that this residue acts as a catalytic base, abstracting a proton from the terminal hydroxyl of the acceptor alcohol, facilitating nucleophilic attack by the activated acceptor on the β-phosphorus of the CDP ( Fig. 7a ). Following either an associative or dissociative mechanism ( Fig. 7b ) this yields CMP and the phosphodiester product ( Fig. 7c ). We cannot unambiguously determine whether this reaction occurs by an associative mechanism via a pentacoordinate, trigonal bipyramidal transition state or by a dissociative mechanism via a trigonal planar intermediate. A plausible associative mechanism is depicted in Fig. 7 . Although the pKa of an isolated aspartate is too low to act as an efficient catalytic base under physiological conditions, substantial elevation of the pKa of catalytic aspartates has been previously described [22] , particularly in the presence of neighbouring negative charges, as is observed here with the clustering of the four conserved aspartates. A base-catalysed mechanism is supported by the observation that many CDP-APs have alkaline pH optima [23] , [24] . Consistent with the presence of a general acid–base catalyst, rabbit phosphatidylinositol (PI) synthase has an alkaline pH optimum for the forward synthase reaction, while displaying a mildly acidic optimum for the reverse activity [25] . 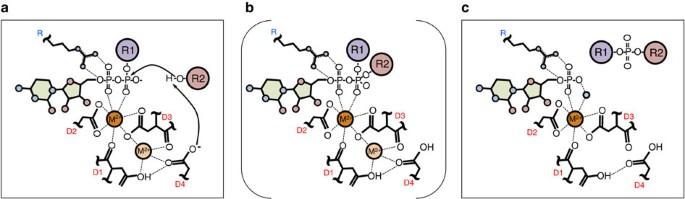Figure 7: CDP-alcohol phosphotransferases effect phosphotransfer by a base-catalysed mechanism. (a) The fourth aspartate in the signature motif, D4, deprotonates the acceptor alcohol (R2, red), activating it for nucleophilic attack upon the beta-phosphorus of the CDP (the pyrimidine ring of which is shown in pale green), to which the donor substituent (R1, purple) is attached by an ester linkage. (b) Here, the transition state of the reaction is shown assuming an associative mechanism proceeding via a penta-coordinate transition state, to yield the product, (c) a phosphodiester linked conjugate of the donor, R1, and the acceptor R2. A water molecule (aqua) replaces the beta-phosphate in coordinating the primary divalent cation. Figure 7: CDP-alcohol phosphotransferases effect phosphotransfer by a base-catalysed mechanism. ( a ) The fourth aspartate in the signature motif, D4, deprotonates the acceptor alcohol (R2, red), activating it for nucleophilic attack upon the beta-phosphorus of the CDP (the pyrimidine ring of which is shown in pale green), to which the donor substituent (R1, purple) is attached by an ester linkage. ( b ) Here, the transition state of the reaction is shown assuming an associative mechanism proceeding via a penta-coordinate transition state, to yield the product, ( c ) a phosphodiester linked conjugate of the donor, R1, and the acceptor R2. A water molecule (aqua) replaces the beta-phosphate in coordinating the primary divalent cation. Full size image The role of the primary divalent cation appears to be to prime the pyro-phosphate for catalysis via an in-line mechanism of substrate transfer, in addition to withdrawing charge from the pyrophosphate, making it more electrophilic and increasing susceptibility to nucleophilic attack. The function of the secondary cation is less obvious. It may contribute to orienting the carboxyl of D 4 appropriately to deprotonate the acceptor. Secondary divalent cation binding sites have also been described for other phosphotransferases, such as cAMP-dependent protein kinase [26] . Strikingly, this mechanism appears to have many common features with that of other phosphotransferases including kinases, which have a completely unrelated fold, but a very similar configuration of active site residues and substrates [27] . A remarkable feature of the CDP-AP family is the chemical diversity of both acceptor and donor substrates. In the active site of the AF2299 structure, in addition to the nucleotide-binding site, we observe two pockets that are likely to host the donor substituent and the acceptor alcohol ( Fig. 4b ). This hypothesis is confirmed for the donor group by our structure showing CDP-glycerol bound to AF2299 ( Fig. 5 ). Given the absolute conservation of residues involved in catalysis and nucleotide binding, the position of the donor and acceptor substrates will most probably also remain constant, so as to allow the reaction to occur. Therefore, the structures reported here are likely to provide a framework in which to investigate the molecular elements underlying substrate specificity. AF2299 appears likely to take inositol-1-phosphate as the acceptor alcohol, an observation that is of particular significance when considered in the context of mycobacterial PI synthesis, which proceeds via a somewhat different pathway to that in other organisms. PI synthases from eukaryotes catalyse the direct formation of phosphatidylinositol from CDP-diacylglycerol (CDP-DAG) and myo-inositol, and they cannot process inositol phosphate [28] . In contrast, mycobacterial phosphatidylinositol is formed in two steps. In the first step, a PI-synthase-like CDP-AP catalyses the conjugation of CDP-DAG with inositol-1-phosphate. Importantly, this enzyme does not recognize inositol, instead specifically recognizing inositol-1-phosphate [29] . This reaction generates phosphatidylinositol-phosphate, which is then processed by a phosphatase of unknown identity to yield phosphatidylinositol. Phosphatidylinositol biosynthesis is a particularly attractive target for the development of anti-tuberculosis therapeutics, as all downstream steps in the synthesis of lipoarabinomannan, an important component of the cell wall, are contingent upon the attachment of mannan chains to a phosphatidylinositol anchor [3] , [30] . The orthogonal substrate specificities of mycobacterial and eukaryotic PI synthases suggest that this may be a feasible avenue for therapeutic intervention. The transmembrane domain of AF2299 shares only 20% identity with M. tuberculosis PI synthase, but the high degree of conservation of specific elements present in AF2299, MT-PI synthases and the DIPP synthases ( Supplementary Fig. 6 ) suggests that AF2299 may provide a useful framework for the design of inositol–phosphate analogues for the inhibition of the mycobacterial PI-synthases. Previous development of inositol-1-phosphate analogues has focused on replacement of the 1-phosphate with an analogous non-hydrolyzable moiety such as phosphonate, but these modifications resulted in inhibitors with significantly lower affinity than the cognate substrate [31] . We would predict that the 1-phosphate interacts with two arginine residues (Arg301 and Arg304 in AF2299), and likely makes a significant contribution to binding affinity, suggesting that alterations at this position are likely to result in reduced affinity. A more productive avenue for exploration may involve replacement of the terminal hydroxyl with a less reactive substituent. The best-characterized role of CDP-APs is in the biosynthesis of phospholipids. In the scheme of this reaction, the lipidic substrate can participate either as a donor substituent, as an acceptor alcohol, or two lipids may act as donor and acceptor respectively. The prokaryotic PGP-synthases and eukaryotic PI-synthases process a lipophilic donor (CDP-DAG) and a polar acceptor, respectively glycerol-3-phosphate [32] and myo-inositol [33] . By contrast, the eukaryotic choline and ethanolamine phosphotransferases that participate in the Kennedy pathway of zwitterionic phospholipid biosynthesis utilize CDP-choline/CDP-ethanolamine as donors, and diacylglycerol as the acceptor alcohol [34] , [35] . Eukaryotic cardiolipin synthases [4] represent a third class in which CDP-DAG condenses with phosphatidyl-glycerol. While representing the first reported structure for any CDP-AP, our current model of AF2299 does not allow us to draw firm conclusions regarding the binding mode of lipid substrates. However, attachment of a bulky, hydrophobic lipid substituent to the β phosphate of CDP would appear to restrict the number of possibilities for the overall disposition of the alkyl chains to only two, of which only one seems plausible. In one orientation, the alkyl chain would project into the polar cavity of the active site towards the acceptor. The more likely scenario, in agreement with the structure of bound CDP-glycerol, has the glycerol moiety of a lipid positioned in the secondary pocket, with the alkyl chains of the lipid exiting into the bilayer between TM2 and TM5. Target identification and cloning A member of the CDP-alcohol phosphatidyltransferase class-I family from Archaeoglobus fulgidus DSM 4304 (AF2299, UniProt accession no. O27985) was identified as a promising candidate for crystallization experiments by the NYCOMPS (New York Consortium on Membrane Protein Structure) high-throughput screening pipeline [36] , [37] . The gene encoding AF2299 was amplified from Archaeoglobus fulgidus DSM 4304 genomic DNA using (5′-tacttccaatccaatgccATGAGGTTAGCGTACGTTAAAAAC-3′) as the forward primer and (5′-ttatccacttccaatgCTAGTTCGTGTAACTTCTGAGTG-3′) as the reverse primer for PCR, where upper case letters indicate gene-specific sequences and lower case letters indicate sequences incorporated into the PCR product that are required for ligation independent cloning. The gene was cloned into the bacterial expression vector pMCSG7-10xHis, introducing an N-terminal decahistidine tag and a TEV protease cleavage site. Protein expression and purification AF2299 was overexpressed in E. coli strain BL21 (DE3) pLysS. Bacterial cultures were grown at 37 °C in 2xYT medium supplemented with 100 μg ml −1 ampicillin and 50 μg ml −1 chloramphenicol. Once the OD 600 reached 1.0, the temperature was reduced to 22 °C, and cells were induced with 0.2 mM isopropyl β-D-1-thiogalactopyranoside (IPTG) after 15 min. After overnight induction at 22 °C, cells were harvested by centrifugation and stored at −80 °C. Cells expressing selenomethionine-substituted protein were grown with a kit containing a minimal medium of M9 salts (M9 SeMET High-Yield Growth Media Kit, Shanghai Medicilon Inc.). A total of 150 mg selenomethionine was added per liter of culture in addition to the selenomethionine provided in the kit. The rest of the protocol was the same as for native protein expression. For large-scale purification of both native and selenomethionine-substituted protein, frozen cell pellets were resuspended in lysis buffer containing 20 mM Na-HEPES (pH 7.5), 200 mM NaCl, 1 mM EDTA, 1 mg ml −1 lysozyme, 20 mM MgSO 4 , 10 μg ml −1 DNase I, 10 μg ml −1 RNase A, 1 mM TCEP, 1 mM PMSF and Complete Mini EDTA-free protease inhibitor cocktail (Roche) as described in the instructions. Cells were lysed with an Emulsiflex C3 homogenizer (Avestin). Lysate was solubilized for 1.5 h with 1% ( w / v ) n-decyl-β-D-maltopyranoside (DM, Anagrade, Affymetrix) in a volume of ~40 ml per cell pellet from 800 ml culture (~6 g). After solubilization, insoluble material was pelleted by ultracentrifugation at 134,000 g for 30 min at 4 °C. Protein was purified by metal-affinity chromatography (Ni-NTA, Qiagen) followed by size-exclusion chromatography (SEC) on a Superose 12 column (GE Healthcare) in a buffer of 20 mM Na-HEPES (pH 7.0), 200 mM NaCl, 0.2% ( w / v ) DM and 1 mM tris(2-carboxyethyl)phosphine hydrochloride (TCEP-HCl). Approximately 1.5 mg of purified protein could be obtained from an 800 ml bacterial culture. Selenomethionine-substituted protein was purified using the same protocol. Crystallization Protein from peak fractions from size-exclusion chromatography was concentrated to 30–35 mg ml −1 (approximated by A 280 nm ) for crystallization using a centrifugal concentrator (Millipore) with a 100 kDa MWCO. Selenomethionine-substituted protein was concentrated to 25–30 mg ml −1 . Crystals were grown at room temperature (20–22 °C) in lipidic cubic phase. Concentrated protein was mixed with monoolein (Sigma) in a 1:1.5 ( w / w ) ratio of protein:monoolein. A Mosquito LCP (TTP Labtech) robot was used to dispense a typical volume of 50–100 nl of protein/monoolein mixture onto a 96-well glass plate, which was covered with 750–1,000 nl precipitant solution and sealed with a glass cover slip. Glass sandwich plates were stored in a 22 °C incubator. Largest crystals grew to ~10 × 30 × 100 μm 3 in 1–2 days in (a) 14–20% ( v / v ) PEG 550 MME, 0.1 M Na-HEPES or Tris–HCl (pH 7.0–8.0), 0.2 M lithium sulphate (CMP/apo structure) (b) 25–30% ( v / v ) PEG 400, 0.1 M Na-HEPES (pH 7.0–7.5), 0.2 M potassium sodium tartrate (CDP structure) or (c) 15% PEG 550 MME, 0.1 M Na-HEPES (pH 7.0), 0.2 M potassium sodium tartrate, 2.5 mM CDP-glycerol and 1 mM TCEP (CDP-glycerol structure). Crystals of selenomethionine-substituted protein grew in similar conditions. A tungsten carbide glass-cutter (Hampton Research) was used to cut and remove the glass cover slip, and crystals were harvested using 20–100 μm MicroLoops and MicroMounts (MiTeGen). Crystals were flash-cooled directly in liquid nitrogen without additional cryoprotection. Diffraction data collection and processing Diffraction data were collected on NECAT beamlines 24-ID-C and 24-ID-E at the Advanced Photon Source (Argonne, IL, USA). Crystals were centred by diffraction, rastering across a grid in one orientation, and then along the orthogonal axis intersecting the position where the best diffraction was obtained in the first orientation. All diffraction data were indexed, integrated scaled using XDS and XSCALE [19] , [38] . Data sets collected above the Se K-edge from two selenomethionine-substituted crystals were used for structure solution by anomalous diffraction methods. Selenium sites were located using SHELXD [39] , [40] , and refined in SHARP [41] . Density modification, including solvent flattening, histogram matching and twofold non-crystallographic symmetry averaging were performed using DM to give an initial experimentally phased electron density map [42] . Model building and refinement An initial model was built using BUCCANEER [43] . The model was manually completed using COOT and refined using the PHENIX crystallographic software package, alternating between cycles of manual building in COOT [44] and refinement in PHENIX [45] . Local torsion angle NCS restraints were employed throughout refinement. Riding hydrogens were included in the last round of refinement. The quality of the model was analysed using the validation module of the PHENIX package, which incorporates Molprobity clash score, density correlation and rotamer analysis [46] . Data collection, refinement and validation statistics for both structures are provided in Table 1 . Protein structure figures were prepared using UCSF Chimera [47] . Within the crystal, the protein packs as stacks of two-dimensional sheets ( Supplementary Fig. 7 ). Within each layer, adjacent dimers are arranged in an up–down orientation, such that the N-terminal domains of adjacent layers in the stack are interdigitated. A stereo figure of representative electron density for the CMP/apo structure and a C-alpha trace depicting the fold is given in Supplementary Fig. 8 . Table 1 Data collection and refinement statistics. Full size table Ca and Mg measurements Ca and Mg measurements were conducted using a dual flame/graphite furnace Atomic Absorption Spectrometer AAnalyst 800, manufactured by Perkin Elmer. Data were collected and processed with WinLab32 software. Ca and Mg concentrations were determined at wavelengths of 422.7 nm and 285.2 nm, respectively, using an air–acetylene flame and standard nebulizer with flow spoiler. Detection limits were 0.02 mg ml −1 and 0.003 mg ml −1 for Ca and Mg, respectively. Each run included calibration with three standards, as well as quality control samples with known concentrations of Ca and Mg. Calibration standards were made in 1% ( v / v ) HCl. All other samples were diluted in 1% ( v / v ) HCl. Duplicate samples of AF2299 at a concentration of 40 mg ml −1 were analysed, as well as a control sample of protein-free buffer. Raw data and derived results are reported in Supplementary Table 2 . How to cite this article: Sciara, G. et al . Structural basis for catalysis in a CDP-alcohol phosphotransferase. Nat. Commun. 5:4068 doi: 10.1038/ncomms5068 (2014). Accession codes: Coordinates and structure factors have been deposited in the Protein Data Base under accession codes 4O6M (CMP/apo), 4O6N (CDP), 4Q7C (CDP-glycerol).